Sex ratio biases in termites provide evidence for kin selection Inclusive fitness theory, also known as kin selection theory, is the most general expansion of Darwin's natural selection theory. It is supported by female-biased investment by workers in the social Hymenoptera where relatedness to sisters is higher than to brothers because of haplodiploidy. However, a strong test of the theory has proven difficult in diploid social insects because they lack such relatedness asymmetry. Here we show that kin selection can result in sex ratio bias in eusocial diploids. Our model predicts that allocation will be biased towards the sex that contributes more of its genes to the next generation when sex-asymmetric inbreeding occurs. The prediction matches well with the empirical sex allocation of Reticulitermes termites where the colony king can be replaced by a queen’s son. Our findings open broad new avenues to test inclusive fitness theory beyond the well-studied eusocial Hymenoptera. Inclusive fitness theory predicts that by investing more resources in certain close relatives, an individual can maximize the transmission rate of its own genes to the next generation via reproduction by kin [1] . The most successful demonstration of this is sex-biased investment in haplodiploid eusocial insects, where the life-for-life relatedness of a worker to her sisters is higher than to her brothers [2] , [3] . Because of this relatedness asymmetry, workers are predicted to invest more resources in sisters than in brothers. Such sex-biased investment has been reported in many empirical studies, providing some of the strongest support for inclusive fitness theory [4] , [5] , [6] , [7] , [8] , [9] . In eusocial diploids, relatedness asymmetries are generally thought to be absent. Therefore, kin selection is predicted not to bias the sex investment ratio in social diploids including termites. While Fisher’s principle explains why the sex allocation ratio of most organisms is 1:1, several mechanisms have been proposed to account for cases in which there is significant deviation from an even sex ratio [10] , [11] . The known mechanisms causing adaptive sex ratio bias includes relatedness asymmetry in social Hymenoptera [2] , [3] , [4] , [5] as mentioned above; genetic interference between sexes such as local mate competition (LMC) [12] , local resource competition [12] , [13] and local resource enhancement [12] , [14] ; inbreeding in haplodiploid insects [15] , [16] ; and differences in the number of breeding seasons between sexes in multi-voltine species [17] , [18] . In this paper, we propose a new mechanism for sex ratio bias via kin selection in diploid social insects. We develop a mathematical model showing that sex-asymmetric inbreeding can cause sex ratio biases. To test the model’s prediction, we compare sex allocation of Reticulitermes termites with different reproductive systems. As predicted by the model, the empirical data show that species with asexual queen succession (AQS; where the original queen is replaced by multiple parthenogenetically produced daughter queens) biases sex allocation toward females, whereas species without AQS show no bias. Model life history Suppose a eusocial insect with sterile workers where some (alate) reproductives specialize on dispersal and founding new colonies and other (non-dispersal) reproductives stay in the natal nest to breed. All reproductive individuals thus contribute to producing new generations of dispersing reproductive, but the number of generations of breeding in the same colony varies from one to several ( Fig. 1a ). In such species sex-asymmetric inbreeding (for example, mother–son and uncle–niece matings) may occur, resulting in male and female founders being unequally efficient as vehicles for genetic contributions to future generations ( Fig.1b ). If sex-asymmetric inbreeding is common, this should lead to biased sex ratios in favour of the parental sex with the greater genetic contribution. 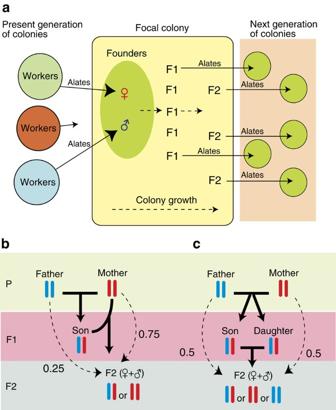Figure 1: Schematic view of sex-asymmetric inbreeding. (a) The typical eusocial breeding system for sex-asymmetric inbreeding. Monogamous founding pairs produce outbred F1 offspring but inbred F2 offspring as the colony grows and both may contribute to founding the next generation of colonies. (b) Mother–son inbreeding resulting in sex-asymmetric genetic contributions, where F2 individuals inherit 0.75 maternal genes and 0.25 paternal genes. (c) Full-sib inbreeding resulting in sex-symmetric genetic contributions, where the grandoffspring (F2) inherit 0.5 maternal genes and 0.5 paternal genes. Figure 1: Schematic view of sex-asymmetric inbreeding. ( a ) The typical eusocial breeding system for sex-asymmetric inbreeding. Monogamous founding pairs produce outbred F1 offspring but inbred F2 offspring as the colony grows and both may contribute to founding the next generation of colonies. ( b ) Mother–son inbreeding resulting in sex-asymmetric genetic contributions, where F2 individuals inherit 0.75 maternal genes and 0.25 paternal genes. ( c ) Full-sib inbreeding resulting in sex-symmetric genetic contributions, where the grandoffspring (F2) inherit 0.5 maternal genes and 0.5 paternal genes. Full size image Sex-asymmetric inbreeding is expected to occur in eusocial insects whenever the following three conditions are met: (i) A colony is founded by a monogamous pair (one male and one female), (ii) deceased founders are replaced by full-sib reproductive offspring in the nest, resulting in inbreeding among the new cohort of reproductives, and (iii) there is a sex-specific difference in longevity between male and female founders, such that either the male or female consistently outlives its partner and inbreeding occurs between parent and offspring, that is inbreeding is sex-asymmetric. Recently, a novel breeding system called AQS has been described in two species of subterranean termites— Reticulitermes speratus [19] and Reticulitermes virginicus [20] —that meet all three of these conditions. Termite colonies are typically founded by a monogamous pair of primary reproductives (adult winged forms), one king and one queen. In Reticulitermes termites, neotenics (also called secondary reproductives or supplementary reproductives) are produced from within the colony upon the death of the primary king and/or queen [21] , [22] . As colonies develop, neotenic queens may differentiate even under the presence of reigning queens to supplement egg production according to the labour needs of the colony. Neotenic individuals can differentiate from either nymphs to become ‘nymphoid’ reproductives with wing pads or from workers to become ‘ergatoid’ reproductives without wing pads ( Fig. 2 ). 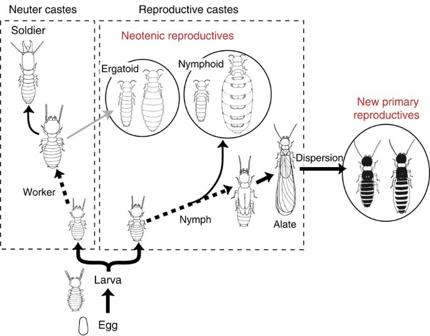Figure 2 Differentiation pathways of primary and neotenic reproductives in the genusReticulitermes. Figure 2 Differentiation pathways of primary and neotenic reproductives in the genus Reticulitermes . Full size image In the subterranean termites R. speratus and R. virginicus , queens produce their neotenic replacement reproductives asexually but use normal sexual reproduction to produce other colony members [19] , [20] . These species undergo typical colony founding by a pair of primary reproductives. Relatively early in the colony life cycle, the primary queen is replaced by numerous secondary queens (female neotenics) that are produced asexually by the primary queen ( Fig. 3a ). These neotenic queens mate with the primary king and produce workers, soldiers and new primary reproductives through sexual reproduction. On the other hand, primary kings live much longer than primary queens. This AQS system enables founding queens to increase their reproductive output while retaining the same transmission rate of their genes to future generations [19] , [20] , [23] ( Fig. 3b ). Therefore, the founder queen can be considered genetically immortal until the colony dies, because female neotenics are themselves replaced by new cohorts of parthenogenetically produced neotenics. When the founder king dies, he can be replaced by a secondary king that is the son of the founder queen and king, effectively resulting in mother–son inbreeding. AQS colonies with a secondary king should thus be expected to bias sex allocation because their inbreeding is sex asymmetric, and we expect that female bias will be more pronounced when the frequency of mother–son inbreeding is higher. 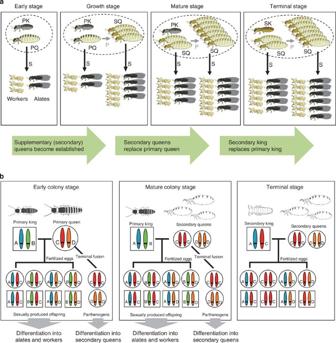Figure 3: Schematic diagram of asexual queen succession as found in someReticulitermestermites. (a) Life history of the species with asexual queen succession (AQS). PK, primary king; PQ; primary queen; SQ, secondary queen; P, parthenogenesis; S, sexual reproduction. (b) Genetic scheme for the breeding system with AQS. Queens are able to reproduce sexually and also asexually. Offspring produced by sexual reproduction develop into workers, soldiers and alates, whereas those produced by parthenogenesis (automixis with terminal fusion) exclusively differentiate into female neotenics and supplement or replace the older queens. Secondary queens also produce the next replacement queens by parthenogenesis. Thus, the primary queens retain their genetic contribution to the next generation even after their death. Squares indicate males and circles indicate females. Figure 3: Schematic diagram of asexual queen succession as found in some Reticulitermes termites. ( a ) Life history of the species with asexual queen succession (AQS). PK, primary king; PQ; primary queen; SQ, secondary queen; P, parthenogenesis; S, sexual reproduction. ( b ) Genetic scheme for the breeding system with AQS. Queens are able to reproduce sexually and also asexually. Offspring produced by sexual reproduction develop into workers, soldiers and alates, whereas those produced by parthenogenesis (automixis with terminal fusion) exclusively differentiate into female neotenics and supplement or replace the older queens. Secondary queens also produce the next replacement queens by parthenogenesis. Thus, the primary queens retain their genetic contribution to the next generation even after their death. Squares indicate males and circles indicate females. Full size image Description of the model Let g f and g m be the proportion of genes in alates derived from the founder female and founder male, respectively. Then, in cases of mother–son mating, the pair producing the F2 offspring consists of the P mother (founder female) and her F1 son ( Fig. 1b ). Under this mating system g f =0.75, but g m =0.25 so that females contribute three times as many genes as males. In contrast, inbreeding through full-sib matings does not result in such sex-asymmetric genetic contributions, as diploid male and female founders would continue to contribute equally to the gene pool of the next generation of alates, that is, g f = g m =0.5 ( Fig. 1c ). Thus, not all types of inbreeding result in sex-asymmetric genetic contributions. To consider the effect of sex-asymmetric inbreeding on sex allocation, let c m and c f be the class reproductive values of male and female founders, respectively. Class reproductive value describes the expected proportion of genes contributed by a class of individuals to a future generation [24] , [25] . When there are n types of mating that occur over the lifespan of the colony (for example, mating between parental founders, mother–son inbreeding, father–daughter inbreeding, so on. ), the class reproductive value of male and female founders, c m and c f , are where sex is either male (m) or female (f), and p i and g sex ,i are the proportion of progeny and the genetic contribution by a founder to the i th-mating type, respectively. Assuming a large enough population in which individuals allocate resources to (invest in) female alates in proportion s , the fitness of a mutant individual who invests in female alates at s * is to determine the ESS (evolutionarily stable strategy) proportion of females, we take the derivative of W with respect to s* , and set the value equal to zero: which gives the solution where the sum of c f and c m is unity, so that the ESS proportion of females is s *= s = c f . Thus, the ESS is in the case where all alates are produced only by mother–son inbreeding, g f =0.75 ( Fig. 1b ) and p i =1, the resulting s =1.0 × 0.75=0.75. When the proportions of alates produced by mother–son inbreeding ( g f =0.75) and outbreeding ( g f =0.5) are p and 1− p , respectively, the resulting proportion of females is given by Empirical test We found that replacement of the primary king by a secondary king happens in the later stages of colony maturity in R. speratus ; of 43 colonies, in which kings were recovered, 40 had a single primary king and three had a single secondary king. All of the neotenic reproductives were nymphoid (male neotenics: N =3; female neotenics: N =3,450). In contrast, previous studies indicate that R. virginicus appears to experience king replacement in an earlier stage of colony establishment, so that 40% of colonies are estimated to have a primary king and 60% a secondary king [20] . We can therefore make the following two predictions concerning the sex allocation in Reticulitermes species: sex allocation in species with AQS will be significantly female biased, whereas sex allocation in species without AQS will not be biased; sex allocation in R. virginicus should be more female biased than in R. speratus . We compared sex allocation in two termite species with AQS ( R. speratus and R. virginicus ) with that of three congeners without AQS ( R. flavipes , R. okinawanus and R. yaeyamanus ). As predicted by our model, the AQS and non-AQS species showed significant differences in the proportion of alate females produced (generalized linear models , AQS versus non-AQS: likelihood ratio x 2 =30.32, d.f.=1, P <0.0001; species: x 2 =4.90, d.f.=3, P =0.18) and in proportional investment in females (AQS versus non-AQS: x 2 =29.13, d.f.=1, P <0.0001; species: x 2 =3.28, d.f.=3, P =0.35; Fig. 4 ). The mean proportion of females in R. speratus was 0.562 (±0.017SE), which was significantly skewed towards females (two-tailed t -test, N =107 colonies including 14,445 individuals, t =−3.476, P <0.001). When adjusted for biomass, the proportional investment was even more female biased (0.587±0.017SE; t =−4.491, P <0.0001; Fig. 4 ), because female alates are larger than males from the same nest. Similarly, the mean proportion of females in R. virginicus was 0.642 (±0.060SE), which was significantly skewed toward females ( N =16 colonies including 5,620 individuals, t =−2.369, P <0.05). Again, there was greater bias in proportional investment in females (0.655±0.059SE; t =−2.585, P <0.05; Fig. 4 ). We also predicted that sex allocation in R. virginicus would be more female biased compared to R. speratus , as there appears to be a higher proportion of secondary kings and thus a higher percentage of mother–son matings in the former species (estimated at 60% in R. virginicus [20] compared to 7% in R. speratus , a significant difference according to Fisher’s exact probability test, P <0.05). Although we did find that R. virginicus had a greater proportional investment in females than R. speratus (0.655 versus 0.587), this difference was marginally non-significant (one-tailed t -test, t =1.38, d.f.=121, P =0.085). The outcome of this direct test on the two AQS species where we did expect a difference in female bias is thus somewhat more encouraging than the overall 'species' test given above, and might reach significance if the limited sample size in R. virginicus ( N =16) could be expanded. 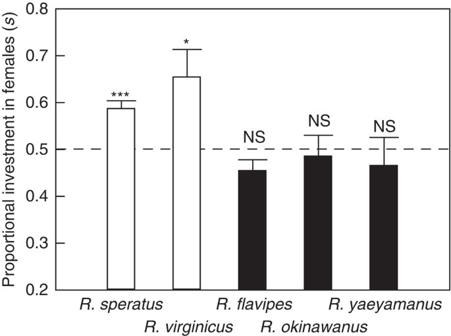Figure 4: Comparison of the observed proportional investment in female alates between species with and without AQS. The species with AQS areR. speratus(N=107 colonies) andR. virginicus(N=16) and those without AQS areR. flavipes(N=43),R. okinawanus(N=11) andR. yaeyamanus(N=7). The AQS species (open bars) showed significantly female-biased investment in comparison with non-AQS species (closed bars) (GLM,P<0.0001). Error bars indicate standard errors. The statistics on the bars indicate the significance level of the deviation from equal allocation (two-tailedt-test: ***P<0.001; *P<0.05). Figure 4: Comparison of the observed proportional investment in female alates between species with and without AQS. The species with AQS are R. speratus ( N =107 colonies) and R. virginicus ( N =16) and those without AQS are R. flavipes ( N =43), R. okinawanus ( N =11) and R. yaeyamanus ( N =7). The AQS species (open bars) showed significantly female-biased investment in comparison with non-AQS species (closed bars) (GLM, P <0.0001). Error bars indicate standard errors. The statistics on the bars indicate the significance level of the deviation from equal allocation (two-tailed t -test: *** P <0.001; * P <0.05). Full size image In contrast, the mean proportion of females in R. flavipes was 0.442 (±0.022SE), which was significantly male- biased ( N =43 colonies including 7,782 individuals, t =2.63, P <0.05), and the proportional investment in females was 0.455 (±0.023SE), which was not significantly different from 0.5 ( t =1.94, P =0.059; Fig. 4 ). Similarly, the mean proportion of females in R. okinawanus was 0.460 (±0.043SE), and neither this ( N =11 colonies including 1353 individuals, t =0.939, P =0.370) nor the proportional investment in females (0.486±0.044SE; t =0.315, P =0.759; Fig.4 ) was significantly different from 0.5. As in R. flavipes and R. okinawanus , the mean proportion of females in R. yaeyamanus was 0.434 (±0.060SE), and neither this ( N =7 colonies including 1,184 individuals, t =1.10, P =0.314) nor the proportional investment in females (0.466±0.061SE; t =0.563, P =0.594; Fig. 4 ) deviated significantly from equality. Based on relatedness asymmetries attributed to haplodiploidy, sex ratio studies of social Hymenoptera have provided the most successful tests of inclusive fitness theory [2] , [3] , [4] , [5] , [6] , [7] , [8] , [9] . Our study shows that diploid genetic system can also generate sexual asymmetry in reproductive values (gene transmission rates) in diploid eusocial colonies with parent–offspring mating. Our model successfully predicted interspecific variation in sex ratio patterns in diploid termites just as the Trivers and Hare hypothesis [2] did for the eusocial Hymenoptera. Sex allocation was indeed more female biased in the two Reticulitermes species with the AQS system than in the three species without AQS. Most recently, the AQS system was also reported in an Italian species Reticulitermes lucifugus [26] , as predicted previously based on highly female-biased sex ratios [23] . In fact, R. lucifugus was found to have a female biased sex ratio, while the sympatric non-AQS species Reticulitermes urbis had an even sex ratio [26] . The preliminary data for these Italian species provide strong support for our model and show how kin selection can be an important force shaping the evolution of sex allocation in diploid eusocial species. In this paper, we predicted more female-biased sex allocations in R. virginicus than in R. speratus, because it is known that R. virginicus experiences king replacement in an earlier stage of colony establishment. So far, however, we do not have enough data to determine how many rounds of king replacement occur in the life of a typical colony. Our model demonstrated that even a single replacement of the king can bias alate sex ratios. If successive king replacement occurs multiple times in the life of a colony, the genetic contribution of a primary queen to the next generation becomes much greater than that of a primary king, resulting in an even more biased sex allocation towards females. After the second replacement of the king, for example, the genetic contribution of a founder female will be g f =0.875 and that of a founder male will be g m =0.125. Future studies of the detailed reproductive schedules in the colony life cycle of these species would enable more quantitative predictions and tests. Our proposed mechanism leading to biased sex ratios is distinctly different from the previously described mechanisms, such as LMC, local resource competition, and local resource enhancement. In these mechanisms, sex-specific competition or its opposite of synergistic enhancement are the only necessary conditions for biased sex ratios [12] , [13] , [14] . Although inbreeding often occurs in species with LMC, the effect of LMC itself is independent of inbreeding [15] , [16] . However, the necessary condition for the present theory is not sex-specific competition or enhancement, but a specific type of inbreeding. In haplodiploids, it is known that inbreeding enhances the effect of LMC on sex ratio bias because an inbred mother is more related to her daughters than she is to her sons [15] , [16] . This mechanism is unique to haplodiploid systems and does not occur in diploid systems. The number of reigning kings and queens in a colony is highly asymmetric in Reticulitermes termites. In all mature colonies of R. speratus , for example, a single primary king or a single secondary king was present, but primary queens had been replaced by an average of 62.37 (±8.54SE) secondary queens. This sex ratio bias of reigning reproductives could be explained by LMC, where a single king can ensure a sufficient supply of sperm to the multiple queens within a colony. However, the LMC biasing the sex ratios of reigning reproductives cannot bias the sex ratios of alates because the nurse workers (actors) gain no benefit from investing more in female alates than in male alates without sex-asymmetry in class reproductive value. Indeed, LMC of neotenic reproductives is common for all Reticulitermes species investigated for which data are present [21] , including some in this paper, but non-AQS species showed equal sex allocations in alates. Another major mechanism for biased sex ratios is relatedness asymmetry in the eusocial Hymenoptera [2] , [3] , [4] , [5] . In halictid bees, the degree of relatedness asymmetry is different between colonies with founding queens and colonies in which the queens are dead and replaced by daughters resulting in split sex ratios between the two types of colonies [27] , [28] , [29] . In addition, worker laying of male eggs in the eusocial Hymenoptera affects relatedness asymmetry and influences sex allocation [30] . However, unlike relatedness asymmetries arising from haplodiploidy, sex-asymmetric inbreeding does not result in asymmetries of relatedness between workers and male or female alates so that there is no conflict over sex allocation between any pairs of colony members. Importantly, in species with sex-asymmetric inbreeding our model predicts all colonies should invest in the same optimal sex allocation and thus no split sex ratio should occur because the class reproductive value of each sex is shared by all colonies. Therefore, the mechanism outlined here is fundamentally different from the mechanism that causes relatedness asymmetries in eusocial haplodiploids. Another proposed, but not confirmed, mechanism for biased sex ratios is the differential breeding tenure between sexes, such as partial bivoltinism, that results in seasonal sex ratio variation [17] , [18] . This mechanism is different from the current model, as inbreeding is not necessary for biased sex ratio to occur. Another model, the haystack model applies to organisms that have local breeding patches with alternating breeding and dispersal [31] , [32] . Selection favours individuals with high reproductive rates during the reproductive stage because such individuals can produce larger numbers of dispersing individuals than those with low reproductive rates. Under this model, a female-biased sex ratio in the reproductive stage is selected to ensure a higher lineage growth rate. Our model is similar to the haystack model in which dispersal and reproductive stages appear alternately. However, mating before dispersal from the natal colony is a necessary condition to bias the sex ratio of dispersing individuals under the haystack model [31] , [32] , whereas it is not in our model. Compared to the eusocial Hymenoptera, little attention has been given to the sex ratios of termites as possible tests of inclusive fitness theory. Unequal sex ratios of dispersing alates are known in several species [33] , [34] . So far, however, there is no good explanation for the large variation in sex allocation ratios in termites, although a few hypotheses have been unsuccessfully proposed to address this phenomenon [35] . Considering the fact that the AQS system was found in termites only very recently and that few species have been the subject of detailed studies of their breeding system, it would not be surprising to see that such a system is more widespread within the Rhinotermitidae and possibly also in other termite families. Given the power of the sex-asymmetric inbreeding model to successfully predict interspecific sex allocation variation among Reticulitermes species, this model may help explain sex ratio variation more generally in termites. The theoretical framework and empirical support presented here provide new opportunities for testing inclusive fitness theory and for understanding the selection forces leading to biased sex ratios. Alate sex ratios We collected 123 colonies of R. speratus in Kyoto and Okayama, Western Japan. Sixteen colonies of R. virginicus and 11 colonies of R. flavipes were collected in Houston and Conroe, Texas, USA. Thirty-two partial colonies of R. flavipes were collected in Massachusetts, USA. Eleven colonies of R. okinawanus were sampled from the main island of Okinawa. Seven colonies of R. yaeyamanus were collected at Ishigaki Island and Iriomote Island, Okinawa prefecture. Each collection was at least 30 m apart from the nearest sampled colony to ensure sampling of different colonies. We examined the proportion of females and the proportional investment in females. Termites were frozen and counted by caste and sex. Sex was determined from the configuration of the caudal sternites [36] . The proportion of females for each colony was evaluated as the number of female alates divided by the total number of alates. To estimate biomass proportion of females as an index of proportional investment in females, 20 alates (or alate nymphs) of each sex were randomly chosen from each colony and dried to constant weight for 24 h in a 60 °C oven. They were then weighed individually to the nearest 0.01 mg (if fewer alates were obtained, all were weighed). The data for numerical and biomass proportion of females were analysed with logistic regression analyses in generalized linear models with the logit link function using reproductive systems (AQS or non-AQS) and species as clustering factors. The species were nested within the reproductive systems. The sex allocation data of each species were also compared to equal allocation by two-tailed one-sample t -tests after arcsine-square-root-transformation. The analyses were made by using the statistical software JMP 8.0.2 (SAS Institute Inc., Cary, NC, USA). Collection of reproductives To obtain reproductives from a sufficient number of natural R. speratus colonies, we collected more than 860 nests in the field. We successfully found the royal chambers, where reproductives and young brood were protected, in 43 colonies. Like many other subterranean termites, Reticulitermes termites are classified as multiple-site nesters based on their nesting and feeding habits, where multiple food sources are interconnected by belowground tunnels and aboveground shelter tubes. Each colony has only a single reproductive centre consisting of several royal chambers and nursery chambers in a single piece of wood, where a king and multiple secondary queens are living together, although the location of the chambers may change over time. After finding young larvae and eggs, which indicate the presence of royal chambers nearby, we removed the parts of the nest wood containing the royal chambers using a chain saw, and then brought them into the laboratory for further dismantling. All reproductives were sampled by cutting the wood into ~15-cm-thick cross-sections, and carefully splitting the wood along the growth rings to expose termites inside. The reproductives from each colony were immediately preserved in 100% ethanol with nestmate workers and nymphs in a vial for subsequent genetic analysis. We distinguished primary reproductives (alate-derived) from secondary reproductives (neotenics) on the basis of the fully melanized body colour and the presence of wing scales. Sex was determined from the configuration of the caudal sternites under a stereoscope. Neotenic reproductives were investigated for the presence or absence of wing pads to separate into nymphoid (nymph-derived) and ergatoid (worker-derived) reproductives. How to cite this article: Kobayashi, K. et al. Sex ratio biases in termites provide evidence for kin selection. Nat. Commun. 4:2048 doi: 10.1038/ncomms3048 (2013).